The evolution and pathogenic mechanisms of the rice sheath blight pathogen Rhizoctonia solani is a major fungal pathogen of rice ( Oryza sativa L. ) that causes great yield losses in all rice-growing regions of the world. Here we report the draft genome sequence of the rice sheath blight disease pathogen, R. solani AG1 IA, assembled using next-generation Illumina Genome Analyser sequencing technologies. The genome encodes a large and diverse set of secreted proteins, enzymes of primary and secondary metabolism, carbohydrate-active enzymes, and transporters, which probably reflect an exclusive necrotrophic lifestyle. We find few repetitive elements, a closer relationship to Agaricomycotina among Basidiomycetes, and expand protein domains and families. Among the 25 candidate pathogen effectors identified according to their functionality and evolution, we validate 3 that trigger crop defence responses; hence we reveal the exclusive expression patterns of the pathogenic determinants during host infection. The soilborne Basidiomycete fungus Rhizoctonia solani (teleomorph: Thanatephorus cucumeris ) is a complex with more than 100 species that attack all known crops, pastures and horticultural species. R. solani is divided into 14 anastomosis groups (AG1 to AG13 and AGBI) [1] . Among R. solani AG1 containing three main intraspecific groups (ISG), the subgroup AG1 IA is one of the most important plant pathogens, which causes diseases such as sheath blight, banded leaf, aerial blight and brown patch [1] , [2] , [3] in many plants, including more than 27 families of monocots and dicots. As the agent of rice sheath blight, R. solani AG1 IA was thought to be mainly an asexual fungus on rice ( Oryza sativa L. ), although sexual structures from its teleomorph ( T. cucumeris ) have been occasionally observed in fields. In nature, R. solani AG1 IA exists primarily as vegetative mycelium and sclerotia ( Supplementary Fig. S1 ). Each year, the blight causes up to a 50% decrease in the rice yield under favourable conditions around the world [4] , [5] . In Eastern Asia, it affects ~15–20 million ha of paddy-irrigated rice and causes a yield loss of 6 million tons of rice grains per year [5] . R. solani AG1 IA is also considered to be the most destructive pathogen for other economically important crops, including corn ( Zea mays ) [3] , [6] and soybean ( Glycine max ) [2] , [7] . Highly resistant rice and corn cultivars have not been found for use in breeding, but quantitative resistance exists [8] . Until now, control strategies have relied mainly on fungicides. Despite the high worldwide rice yield losses caused by R. solani AG1 IA, only limited information is available about the genetic structure of its populations and reproductive mode [5] , [9] . The main objective of our study was to elucidate the possible molecular basis of host–pathogen interactions and pathogenic mechanisms of the rice-infecting pathogen R. solani AG1 IA, which could provide knowledge for improving the yield of food crop in agriculture. Genome sequencing and analysis We used a whole-genome shotgun (WGS) sequencing strategy and the Illumina Genome Analyser (GA) sequencing technology. A 36.94-Mb draft genome sequence was assembled using the high-quality sequenced data ( Supplementary Table S1 ) and SOAPdenovo [10] . 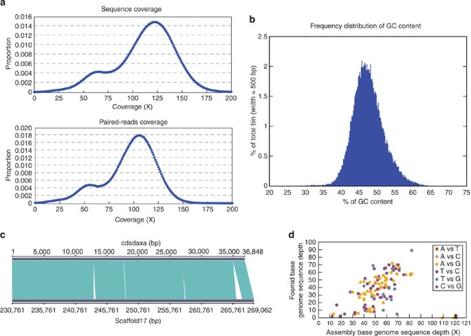Figure 1: Genomic sequence and paired reads coverage. (a) Distribution of genomic coverage (upper) and paired reads coverage (bottom). A major peak was detected at 121 × and 105 × coverage, and a second peak was detected at 66 × and 55 × that showed nearly half of the coverage of the main peak, which indicates highly heterozygous regions that were not merged in the assembly or hemizygous regions. (b) Frequency distribution of GC content. Reads of library with an insert size of 173 bp were used for analysing. Reads were aligned to the assembly using Burrows–Wheeler Aligner42. (c) Comparison of the assembled genome scaffold 17 with a fosmid cdsdaxa sequence. The sequence depth was calculated by mapping the Illumina Genome Analyser short reads with an insert size of 173 bp for the genome assembly10. The remaining unclosed gaps on the scaffolds are marked as white blocks. (d) The sequence depth and a coverage of the genome assembly bases for mismatches of fosmid and genome assembly bases. The N50 sizes of the scaffold and contig were 474.50 Kb and 20,319 bp, respectively ( Table 1 , Fig. 1 ). The G+C content of the genome was 47.61%. The heterozygosity in the R. solani AG1 IA genome was estimated to be 0.12%, and 43,121 SNPs were detected in the assembly. The coding DNA sequences contain 10,489 open reading frames (ORFs) [11] ( Supplementary Note 2 ). Totally, 6,156 genes were annotated, and among these genes 257 genes were assigned to the pathogen–host interaction (PHI) database. Moreover, 2 ribosomal RNAs and 102 transfer RNAs were predicted. Table 1 Description of R. solani AG1 IA genome assembly. Full size table Figure 1: Genomic sequence and paired reads coverage. ( a ) Distribution of genomic coverage (upper) and paired reads coverage (bottom). A major peak was detected at 121 × and 105 × coverage, and a second peak was detected at 66 × and 55 × that showed nearly half of the coverage of the main peak, which indicates highly heterozygous regions that were not merged in the assembly or hemizygous regions. ( b ) Frequency distribution of GC content. Reads of library with an insert size of 173 bp were used for analysing. Reads were aligned to the assembly using Burrows–Wheeler Aligner [42] . ( c ) Comparison of the assembled genome scaffold 17 with a fosmid cdsdaxa sequence. The sequence depth was calculated by mapping the Illumina Genome Analyser short reads with an insert size of 173 bp for the genome assembly [10] . The remaining unclosed gaps on the scaffolds are marked as white blocks. ( d ) The sequence depth and a coverage of the genome assembly bases for mismatches of fosmid and genome assembly bases. Full size image The mitochondrial genome of R. solani AG1 IA assembled as a circular molecule of 146 kb, with an overall G+C content of 33.8%. In all, 21 ORFs were predicted. A total of 26 tRNAs, 1 rRNA and 4 ribozymes were identified. Twenty-nine gaps were finally filled using the PCR technique ( Table 1 , Supplementary Fig. S2 , Supplementary Note 2 ). Indeed, it is the largest mitochondrial genome sequence among fungi thus far. Additionally, we adopted the comprehensive approaches to assess the large-scale and local assembly accuracy of the scaffolds including Sanger protocols ( Fig. 1c , Supplementary Fig. S3 , Supplementary Tables S2 and S3 , Supplementary Note 2 ). It showed that we assembled the diploid multinuclei genome of R. solani AG1 IA, and the assembly was highly accurate. The R. solani AG1 IA repeat content DNA transposons and retrotransposons including 81 families are identified in R. solani AG1 IA, which accounts for 5.27% of the 36.94-Mb genome sequence ( Supplementary Table S4 , Supplementary Note 3 ). Among the repetitive elements, Gypsy comprised 1,189,261 bp and were the most abundant type of transposon elements (TEs). They account for 65.18% of the TEs and 3.43% of the assembly, and when compared with the Gypsy LTR retrotransposons mined from 25 fungal species genomes from Ascomycota and Basidiomycota [12] , more copies were detected in R. solani AG1 IA. Furthermore, tandem repeats of ~55,417 bp were identified. In all, repeat elements were ~5.43% of the assembly. The genome of R. solani AG1 IA showed no evidence of a whole-genome duplication. Among Basidiomycetes, the similarity of repeat contents exists among R. solani AG1 IA, Postia placenta and Cryptococcus neoformans (5% of genome repeats). However, TEs content in the R. solani AG1 IA genome is higher than the content of 2.5% observed in Coprinopsis cinerea and the 1.1% content in Ustilago maydis and is much lower than the 45% content in Melampsora larici-populina , the 43.7% content in Puccinia graminis f. sp. tritici , and the 21% content in Laccaria bicolor of Basidiomycetes. In general, the relatively low repeat content of the R. solani AG1 IA genome is similar to what would be expected for small, rapidly reproducing eukaryotic organisms [13] . We deduce that the R. solani AG1 IA contains DNA methylase genes (AG1IA_00169, AG1IA_00211, AG1IA_01948, AG1IA_05357), which may inhibit repeat element expansion [14] . Evolution and comparative genomics Comparative analyses of the available Basidiomycete genomes show that L. bicolor , P. placenta and rusts M. laricis-populina , P. graminis have more genes ( Supplementary Table S5 ). In all, 608 ortholog groups with only a single gene from each fungus and 102 ortholog groups of nine fungi were predicted, but no M. oryzae groups were found. Among the 102 groups, only a single gene from each fungus was included in the 37 ortholog groups. The genes in these 102 groups were assigned to 426 KOG groups. Not surprisingly, the Basidiomycete groups included many proteins involved in basic cellular processes. However, 33 KOG groups contained proteins that were found in all species of these fungi, which were absent from the of M. oryzae such as Gab-family adaptor protein, protein tyrosine phosphatase. This number of conserved clusters reflects the small evolutionary distance between members of Basidiomycete, as well as complex patterns of gene gains and losses during the evolution of fungi. The differences and quantities of the ortholog groups among the fungi are shown using a Venn diagram ( Fig. 2a ). 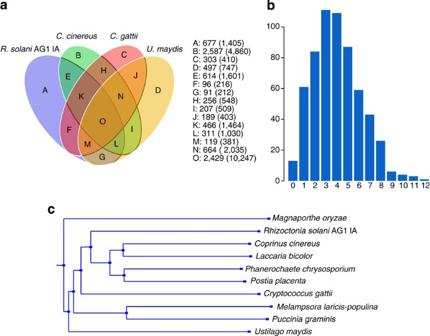Figure 2: Phylogenetic relationship ofR. solaniAG1 IA with other Basidiomycetes fungi and orthologs. (a) Venn diagram showing orthologs between and among the four sequenced Basidiomycete fungi. The values explain the counts of ortholog groups and the counts of genes in parentheses. (b) Distribution of tree branch lengths of 608 single-copy orthologs. The tree branch length of each ortholog group was calculated using codeml with the JTT amino-acid substitution model from the PAML package, based on the CLUSTALW alignment52,53. The branch lengths indicate different evolutionary rates of these ortholog groups. The distribution of the branch length values was determined by the Shapiro–Wilk test (P<0.01). A peak (111 ortholog groups, 18.26%) is distributed near the tree length of 3, and the tree length of 40 ortholog groups (6.58%) was estimated. (c) The phylogeny was constructed using TREEBEST with the neighbour-joining method from 608 single-copy orthologs (each fungus has only one gene in an ortholog group). Protein alignments were analysed using MUSCLE51. Figure 2: Phylogenetic relationship of R. solani AG1 IA with other Basidiomycetes fungi and orthologs. ( a ) Venn diagram showing orthologs between and among the four sequenced Basidiomycete fungi. The values explain the counts of ortholog groups and the counts of genes in parentheses. ( b ) Distribution of tree branch lengths of 608 single-copy orthologs. The tree branch length of each ortholog group was calculated using codeml with the JTT amino-acid substitution model from the PAML package, based on the CLUSTALW alignment [52] , [53] . The branch lengths indicate different evolutionary rates of these ortholog groups. The distribution of the branch length values was determined by the Shapiro–Wilk test ( P <0.01). A peak (111 ortholog groups, 18.26%) is distributed near the tree length of 3, and the tree length of 40 ortholog groups (6.58%) was estimated. ( c ) The phylogeny was constructed using TREEBEST with the neighbour-joining method from 608 single-copy orthologs (each fungus has only one gene in an ortholog group). Protein alignments were analysed using MUSCLE [51] . Full size image The R. solani AG1 IA genes consist of 9,324 families, and of these families, 4,863 are unique, among which 4,538 are single-gene families ( Supplementary Table S5 ). The R. solani AG1 IA undergoing genome reduction display a parallel process of redundancy elimination, by which gene families are reduced to one or a few members with genes family size 1.12. Other large gene families in Basidiomycetes show wider sequence divergence, suggesting they are probably older, and certain functions are overrepresented in large families. We calculated the tree branch length of 608 clusters of the 1:1 orthologs of 10 fungi ( Fig. 2b ). The phylogenetic tree ( Fig. 2c ) confirms R. solani closer relationship to Agaricomycotina among Basidiomycetes. The result may contribute to the resolution of the major problematical nodes in the phylogeny of Basidiomycetes, well resolve the backbone of the Agaricomycotina phylogeny and elucidate the diversity and evolution of the living modes and shifts among hosts. Gene Ontology (GO) term analysis on the important cereal pathogens U. maydis , M. oryzae and R. solani AG1 IA [15] , [16] showed R. solani AG1 IA had unique enriched functional genes, notably an obviously expanded collection of potentially pathogenic GO classifications. Moreover, using Gene Ontology Slim [17] , the largest values for genes were also detected in R. solani AG1 IA ( Supplementary Fig. S4 , Supplementary Note 4 ). The results indicate that the gene function and enrichment among specific types of pathogens evolved independently. At least in part, these differences are likely related to the different parasite lifestyles. The top 100 enriched PFAM domains were depicted for R. solani AG1 IA ( Supplementary Fig. S5a , Supplementary Note 4 ). The large suites of protein domains common in Basidiomycetes but also expanded families with certain GO terms were also revealed ( Supplementary Fig. S5b ). Transcriptome analysis during infection To detect the pathogenicity genes expressed during the entire infection process, the transcriptomes of R. solani AG1 IA at six time points were analysed. In total, we found that 10,103 genes were expressed. From the 18- to 72-h infection stages, specific genes were upregulated, respectively ( Supplementary Fig. S6 ). Comparisons of the relative numbers of upregulated genes in different GO classes revealed the enriched genes were associated with certain GO terms ( Supplementary Fig. S7 ). Among these GO classes, some genes associated with pathogenicity showed a tendency for increased gene number during the host infection process. Meanwhile, other uniquely enriched genes within the GO classes also showed the same expression tendency ( Supplementary Note 5 ). We deduced from the GO annotations that these genes could be related to infection. Although we cannot confirm that these genes are directly related to pathogenesis, we can obtain the trends from this information that can be further evaluated using the transcriptome pattern. Genes involved in pathogenicity Recent studies have demonstrated a strong relationship between the repertoire of carbohydrate-active enzymes in fungal genomes and their saprophytic lifestyle [18] . Comparisons of the phytopathogens revealed that the predicted 223 carbohydrate-active enzymes (CAZymes) in R. solani AG1 IA are only higher than those of the Basidiomycete phytopathogen U. maydis but lower than most of pathogens ( Supplementary Table S6 ). Among the CAZymes, the level of the glycoside hydrolase (GH) family showed a similar trend except P. graminis . However, R. solani AG1 IA had some conspicuously enriched GH and polysaccharide lyase (PL) families ( Supplementary Table S7 ). We found that cellulose and hemi-cellulose-degrading enzymes are also reduced in R. solani AG1 IA ( Supplementary Fig. S8a ). However, R. solani AG1 IA has an expanded set of other cell wall-degrading genes, including pectinase genes, xylanase genes and laccase genes ( Supplementary Fig. S8b , Supplementary Note 6 ). Meanwhile, some putative pathogenic factors such as cutinase genes (CAZyme family CE5) were not predicted. Altogether, our findings reveal that although the necrotrophs have broader host ranges, they do not often express more cell wall-degrading enzymes than biotrophs. The transcripts putatively encoding CAZymes showed differential expression during infection, and 205 transcripts showed a specific expression pattern in six infection stages ( Supplementary Fig. S9 , Supplementary Note 6 ). In total, 122, 156, 133, 110 and 86 CAZyme families were upregulated from the 18- to 72-h stage, respectively, the enriched enzyme transcripts appeared at 24 and 32 h after inoculation ( Fig. 3 , Supplementary Table S8 ). The GH family members and classes involved in infection process showed the trend towards a peak at the 24-h stage. The hemi-cellulose-degrading enzyme transcripts peaking at 24 h, the cellulose and pectin degrading enzyme transcript peaks appearing at 32 and 48 h ( Supplementary Table S9 ). Each GH family member was differentially expressed during the different stages. However, the transcript levels of families in different stages were not consistent with the family numbers. GH72, GH5, GH13, PL4 showed the highest levels, which suggests that these key enzymes have a higher activity and have an important role during host infection ( Fig. 3 , Supplementary Fig. S9 ). The gene expression profiles are distinct at the different infection times, and it is likely that the expression of specific genes encoding degradation-associated enzymes progressively damaged the rice plant during infection. 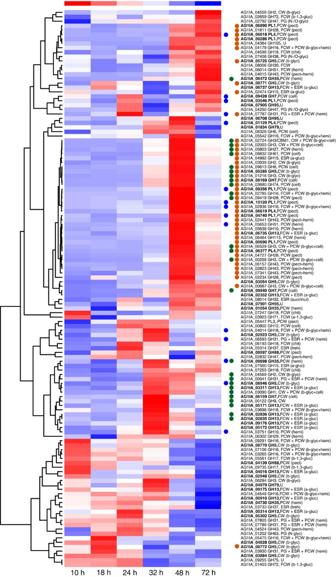Figure 3: The expression pattern of genes coding for the degradative enzymes ofR. solaniAG1 IA. There are totally 114 GH and 12 PL family members expressing in the six infection stages after inoculation (the 10-, 18-, 24-, 32-, 48- and 72-hr stage). The colour scale indicates transcript abundance relative to the mycelium before inoculation: red, increase in transcript abundance; blue, decrease in transcript abundance. The black bold genes are the enriched GH and polysaccharide lyase (PL) transcripts ofR. solaniAG1 IA, compared with the other sequenced pathogens.R. solaniAG1 IA had conspicuously enriched GH and PL families: GH13, GH5, GH95, GH35, GH88, GH7, GH79, PL1 and PL4. Among them, GH13 member α-amylase catalyse the hydrolysis of starch and sucrose in crops. The twofold changes in transcript abundance are marked with circles at the different infection stages; blue, at the 24-h stage; green, at the 32-h stage; dark orange, at the 48-h stage. The enzyme families are defined according to the carbohydrate-active enzyme database. The substrate of CAZy families: CW, cell wall; ESR, energy storage and recovery; FCW, fungal cell wall; PCW, plant cell wall; PG, protein glycosylation; U, undetermined; a-gluc, a-glucans (including starch/glycogen); b-glyc, b-glycans; b-1,3-gluc, b-1,3-glucan; cell, cellulose; chit, chitin/chitosan; hemi, hemicelluloses; inul, inulin; N-glyc, N-glycans; N-/O-glyc, N-/O-glycans; pect, pectin; sucr, sucrose; and treh trehalose. Pearson correlation was used for distance calculations, and the average linkage method was chosen for clustering. Figure 3: The expression pattern of genes coding for the degradative enzymes of R. solani AG1 IA. There are totally 114 GH and 12 PL family members expressing in the six infection stages after inoculation (the 10-, 18-, 24-, 32-, 48- and 72-hr stage). The colour scale indicates transcript abundance relative to the mycelium before inoculation: red, increase in transcript abundance; blue, decrease in transcript abundance. The black bold genes are the enriched GH and polysaccharide lyase (PL) transcripts of R. solani AG1 IA, compared with the other sequenced pathogens. R. solani AG1 IA had conspicuously enriched GH and PL families: GH13, GH5, GH95, GH35, GH88, GH7, GH79, PL1 and PL4. Among them, GH13 member α-amylase catalyse the hydrolysis of starch and sucrose in crops. The twofold changes in transcript abundance are marked with circles at the different infection stages; blue, at the 24-h stage; green, at the 32-h stage; dark orange, at the 48-h stage. The enzyme families are defined according to the carbohydrate-active enzyme database. The substrate of CAZy families: CW, cell wall; ESR, energy storage and recovery; FCW, fungal cell wall; PCW, plant cell wall; PG, protein glycosylation; U, undetermined; a-gluc, a-glucans (including starch/glycogen); b-glyc, b-glycans; b-1,3-gluc, b-1,3-glucan; cell, cellulose; chit, chitin/chitosan; hemi, hemicelluloses; inul, inulin; N-glyc, N-glycans; N-/O-glyc, N-/O-glycans; pect, pectin; sucr, sucrose; and treh trehalose. Pearson correlation was used for distance calculations, and the average linkage method was chosen for clustering. Full size image Fungal pathogens generally produce an array of secondary metabolites, some of which are involved in pathogenesis [19] . We found the 5,655 bp key AROM gene (AG1IA_04890), which participates in the synthesis of PAA, to have 91% identity with the reported R. solani strain [20] . However, we found no homologous hits for the corresponding biosynthetic genes of the other reported mycotoxins in the database [21] against the R. solani AG1 IA genome. Ten secondary metabolite biosynthesis enzymes were identified by SMURF, the NRPS predictor [22] , [23] (one polyketide synthase PKS, four nonribosomal peptide synthetases NRPSs and five prenyltransferases DMATSs) ( Supplementary Table S10 , Supplementary Fig. S10 ). Although these candidate enzymes of R. solani AG1 IA are fewer, the enrichment for DMATs most likely reflects the abundant productions of indole alkaloids [22] . Their unevenly distribution for rapid gene gain and loss was revealed among fungi ( Supplementary Table S11 , Supplementary Note 6 ). The lineage-specific expansions of secondary metabolite synthase genes in R. solani AG1 IA may be responsible for adaptation to its exclusive parasite life. Cytochrome P450s (CYPs) are involved in pathogenesis and the production of toxins [24] . A total of 68 putative CYPs (sixteen families) were identified and clustered in the R. solani AG1 IA genome ( Supplementary Fig. S11a ). Three main categories of expression patterns can be identified during the host infection ( Supplementary Fig. S11b , Supplementary Note 6 ). In all, 187 transporters and 48 ABC transporters are also predicted ( Supplementary Note 6 ). Despite fewer predicted transporter genes [25] , R. solani AG1 IA had the highest number of ABC genes per 1 Mb of genome and exclusive subfamilies likely linked with a unique parasitic lifestyle among Basidiomycetes. The R. solani AG1 IA secretome A subset of secreted proteins from pathogens is expected to determine the progress and success of the infection [26] . The 965 potentially secreted proteins (9.17% of the proteome) of R. solani AG1 IA were analysed by prediction algorithms [27] , [28] ( Supplementary Table S12 , Supplementary Note 7 ). R. solani AG1 IA has a smaller secretome than hemi-biotrophic fungi such as M. oryzae and F. graminearum , but its secretome is larger than most of the biotrophs [29] . Among Basidiomycetes, the rusts and Laccaria have a much larger secretome ( Supplementary Table S12 ). During rice–fungus interaction, 234 secreted proteins showed a twofold or greater difference in expression during the early infection progress ( Supplementary Fig. S12 ). Intriguingly, 103 small cysteine-rich proteins being considered to be potential plant effectors [30] were identified among the predicted secreted proteins. The R. solani AG1 IA candidate effectors and their validation Recent advances revealed the extensive effector repertoires of the pathogens and their functions manipulating host cells. The proteinaceous effectors from necrotrophic fungal pathogens were reported [31] . It has already become clear that the receptors of some necrotrophic effectors operate as dominant disease susceptibility genes [32] . The pathogenicity of R. solani AG1 IA has been studied. However, no effector has been reported before our analysis. We did not identify effectors based on the motifs of reported fungal effectors in our genome [31] , [33] . We found the homologous cyclic peptide synthetases (AG1IA_00102, 3e-39, AG1IA_02283, 8e-14 and AG1IA_07415, 3e-16) that catalyse HC-toxin effector from Cochliobolus carbonum [31] . In addition, four candidate homologous E3 ubiquitin ligase effectors, similar to those in bacterial pathogens, were predicted [34] . To identify the novel potential effectors, we selected 45 twofold or greater upregulated candidate genes encoding secreted proteins for testing ( Supplementary Fig. S12 , Supplementary Note 8 ). The expressed proteins were inoculated into rice, maize and soybean leaves ( Supplementary Fig. S13 ). Interestingly, three classes of potential secreted effectors, AG1IA_09161 (glycosyltransferase GT family 2 domain), AG1IA_05310 (cytochrome C oxidase assembly protein CtaG/cox11 domain) and AG1IA_07795 (peptidase inhibitor I9 domain) caused cell death phenotypes after inoculation at 48 h ( Fig. 4a and Supplementary Fig. S14a ). Meanwhile, these classes showed host-specific toxin characteristics for different hosts (rice, maize and soybean), including 40 different rice cultivars, and caused different degrees of necrosis phenotypes ( Supplementary Fig. S14b ). The glycosyltransferase GT-domain effectors were previously reported in the bacterium Clostridium difficile during a host–bacterium pathogen infection but have not been reported in fungi [35] . A role of inhibitor domain effectors in plant defence has been previously reported in phytopathogens [33] ( Supplementary Note 8 ). However, a peptidase inhibitor I9 domain effector that targets host plants has not been reported to date. In addition, the CtaG/cox11 domain effector is reported for the first time in fungi. Our findings reveal the possibility that there are proteins active in host cells and are delivered by the fungus to trigger a defence response, although the delivery mechanisms for all of these effectors require further investigation. 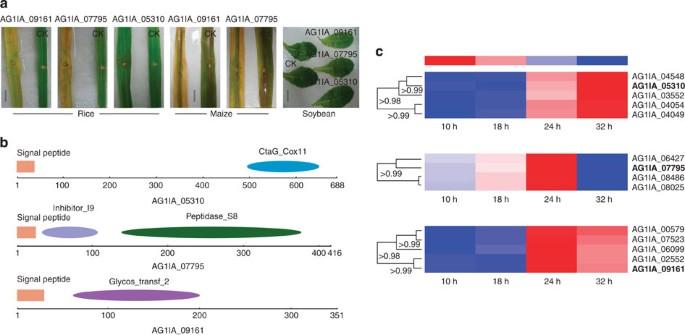Figure 4: Candidate effectors cause necrotic phenotypes in rice, corn and soybean. (a) Phenotypes observed on rice and maize leaves but not observed on soybean leaves. The effectors are encoded by the AG1IA_09161, AG1IA_07795 and AG1IA_05310 genes, respectively, and the cell death phenotypes were visible after inoculation with purified proteins after 48 h. CK represents the total expressed proteins of theE. colistrain harbouring the empty pEASY-TlTM E1 vector. Three replicates of three plants of each line were evaluated for toxin sensitivity. Scale bars (rice), 3 cm; scale bars (maize), 4 cm; scale bars (soybean), 3 cm. (b) Genes with signal peptides (red) and domain structures. CtaG-cox11 domain(blue), peptidase_S8 domain (green), inhibitor I9 domain (light purple) and glycosyltransferase GT family 2 domain (dark purple) are identified in the Pfam database. (c) Clustering of predicted effectors. The hierarchical clustering statistical method based on the Pearson correlation (correlation>0.98) and the average linkage was used. Figure 4: Candidate effectors cause necrotic phenotypes in rice, corn and soybean. ( a ) Phenotypes observed on rice and maize leaves but not observed on soybean leaves. The effectors are encoded by the AG1IA_09161, AG1IA_07795 and AG1IA_05310 genes, respectively, and the cell death phenotypes were visible after inoculation with purified proteins after 48 h. CK represents the total expressed proteins of the E. coli strain harbouring the empty pEASY-TlTM E1 vector. Three replicates of three plants of each line were evaluated for toxin sensitivity. Scale bars (rice), 3 cm; scale bars (maize), 4 cm; scale bars (soybean), 3 cm. ( b ) Genes with signal peptides (red) and domain structures. CtaG-cox11 domain(blue), peptidase_S8 domain (green), inhibitor I9 domain (light purple) and glycosyltransferase GT family 2 domain (dark purple) are identified in the Pfam database. ( c ) Clustering of predicted effectors. The hierarchical clustering statistical method based on the Pearson correlation (correlation>0.98) and the average linkage was used. Full size image Protein effector genes from pathogens have been shown to be undergoing rapid evolution including duplication, diversification, deletions and poit mutations [31] . PCR analysis resulted in 9 positive amplifications on the AG1IA_09161 effector gene from 15 R. solani AG1 IA isolates, corresponding to an average deletion frequency of 40%, and the polymorphs were shown among the different amplicons ( Supplementary Table S13a and Supplementary Fig. S14c ). The strong evidence of positive diversifying selection in the AG1IA_09161 effector gene was confirmed ( Supplementary Table S13b ). Additionally, 20 homologous members from candidate effectors were predicted. However, these genes typically did not encode secreted proteins except AG1IA_03878, AG1IA_07285, AG1IA_09305, AG1IA_09664. So, these four similar domain secreted proteins were also predicted as potential effectors. Indeed, based on the hierarchical clustering method, we identified 18 potential effectors that were grouped into three classes of verified effectors with high Pearson correlation values >0.96 (ref. 36 ). The potential effectors of R. solani AG1 IA are revealed and clustered ( Fig. 4c ). Novel virulence-associated factors in the transduction signal pathway Core elements of the mitogen-activated protein kinase (MAPK) and calcium signalling pathways are required for virulence in a wide array of fungal pathogens [37] . In R. solani AG1 IA, 9 putative G protein subunits ( Supplementary Table S14 , Supplementary Note 9 ) and 13 G-protein-coupled receptors GPCR-like genes were identified ( Supplementary Table S15 ). Notably, three novel Group IV Gpa4 subunits homologous to the one Gpa4 subunit reported in U. maydis [38] were predicted. All of the 13 GPCR-like proteins were predicted and evaluated [30] . However, no GPCR with a specific extracellular membrane spanning the CFEM domain was detected except only four proteins with CFEM domains ( Supplementary Fig. S15 ). This CFEM domain GPCR was actually absent in the Basidiomycete fungi [15] . Thus, because of their lack of a large repertoire of these GPCRs, Basidiomycete pathogens most likely have a reduced ability to react to extracellular signals from environmental stimuli, as compared with Ascomycete pathogens. However, R. solani AG1 IA contains more homologues to Homo sapiens mPR-like GPCRs and pheromone receptors to adapt to the environment, including a NCD3G (AG1IA_09056) nine-cysteine domain ( Supplementary Note 9 ). Moreover, we predicted 22 homologues in the MAPK pathway, 15 homologues in the calcium calcineurin pathway and 5 homologues in the cAMP pathway. Previous studies have shown that field isolates of AG 1, 2, 4 and 8 have a bipolar mating system, in which the heterokaryon formation is controlled by two different factors [39] . However, mating-type ( MAT ) genes have not been identified in T. cucumeris thus far. In Agaricomycetes, the two classes of genes (those encoding pheromone receptors and HD1/HD2 transcription factors) are part of the MAT locus in bipolar systems ( Supplementary Note 10 ). In the R. solani AG1 IA genome, we found the homologous HD1 (AG1IA_06139) and HD2 (AG1IA_08558) sequences to Pleurotus djamor , and we detected similar HD1/HD2 specific domains according to the homologous motifs in Basidiomycetes [40] . In the assembly, we did not find diverged HD1 and HD2 mating type genes, which would be expected in a diploid basidiomycete. Moreover, the arrangement of the B mating type gene cluster was highly conserved in Basidiomycetes. The Ste3-like pheromone receptors (AG1IA_09250, AG1IA_09224 and AG1IA_08458) were predicted, and the other orthologs to the members of the S. cerevisiae MAPK cascade were also detected, including Ste20 (AG1IA_08460, AG1IA_02495), Ste11 (AG1IA_02095), Ste7 (AG1IA_06884), Fus3 (AG1IA_04098, AG1IA_01087) and Ste12 (AG1IA_08474). Based on the previous classic study, the pheromone/receptor pair genes and HD proteins are theoretically physically linked [39] , however, in R. solani AG1 IA assembly, these genes were scattered on the different scaffolds (the scaffold 84, 54, 30, 1, 3 and 4). Among the core elements, Ste12 can also control fungal virulence downstream of the pathogenic MAPK cascade as a master regulator of invasive growth in plant pathogenic fungi [41] . A novel protein Ste12 was detected, which contains two C-terminal C2H2 zinc finger motifs ( Supplementary Fig. S16 , Supplementary Note 9 ). Determining the function of proteins such as Ste12 in the transduction signal pathway during host infection could elucidate the mechanism by which fungal pathogens cause disease in plants in the future. The Rhizoctonia solani represents an important group of soilborne basidiomycete pathogens. Among the phylum Basidiomycota, the complexity of the history of the Agaricomycotina is highlighted. The eight-clade view of Agaricomycete diversity was reflected, and distribution of 14 major clades of Agaricomycetes were identified. However, the studies left many questions and controversies unresolved for lack of explicit phylogenetic analyses. Evolution analysis of sequenced Agaricomycete fungi including R. solani AG1 IA provides the important evidence to support Agaricomycete molecular classification, and confirms firstly the divergent placement of R. solani AG1 IA among Agaricomycotina. As only sequenced plant fungal pathogen in the subphylum, the genome will undoubtedly provide valuable information about the genetic features that distinguish pathogenic and saprophytic lifestyles among the Basidiomycetes. In addition, comprehensive comparisons with the forthcoming genome data from other fungal taxa may yield important clues about their origins and influences on other organisms in the tree of life. Its complex multiple AGs and its multi-nuclear nature have made understanding R. solani evolution previously very difficult. Our study does provide an important advance in this field and will hopefully provide it with the much needed catalyst to develop the necessary tools and resources required to properly begin to understand it. Our analysis of the genome has determined the likely genetic requirements for the necrotrophic phytopathogen to invade and colonize the rice plant. In contrast to previous reports, we conclude that necrotrophy likely does not require a large number of CAZymes and secondary metabolites during host infection, at least for R. solani AG1 IA, which mainly utilizes key pathogenic GHs and genes. Furthermore, secreted proteins could have an important role in pathogenesis. The novel divergent elements, such as Gα proteins, GPCRs in MAPK sigaling pathway, are dedicated to the exclusive parasitic lifestyle and regulate nutrition, reproduction and pathogenicity in the signal transduction pathway. Moreover, 257 genes including the candidate effector (AG1IA_00102) from the R. solani AG1 IA genome were assigned to the PHI database, so we could define the potential pathogenicities of these predcited factors. In addition, among the considerably diverse secreted proteins, novel candidate effectors were found to modulate the host responses and trigger plant cell death. R. solani AG1 IA does not possess simple pathogenic mechanisms that only utilize a battery of lytic and degradative enzymes for infection. We hypothesize that R. solani AG1 IA pathogenesis includes key GHs, secondary metabolites and diverse effectors to suppress the host defences at the early infection stage. HR and the plant defence can then be activated, which is followed by the progressive expression of specific genes encoding degradation-associated enzymes to damage the rice plant during PHIs. Furthermore, the effector genes of R. solani have been shown to undergo rapid evolution [31] . Among the different R. solani AG1 IA isolates and intraspecific groups, different classes of effectors may have undergone rapid evolutionary changes, which may account for the varying virulence of the many AGs, ISGs and isolates of R. solani , as well as their ability to infect a wide range of plants. These different AGs or ISGs provide a species-specific repertoire of effector genes. Furthermore, the infection of rice, maize and soybean by R. solani AG1 IA provides a model of necrotrophic plant interactions. Therefore, the pathogenic mechanism can be elucidated by the intensive study of the genomics and heredity of the crops. In traditional breeding, no crops are highly resistant to Rhizoctonia . Although some resistant quantitative trait loci were found in rice and maize, the cloning and application of resistance genes has not yet been reported. The availability of effectors will allow rice geneticists and breeders to identify and evaluate, in the germplasm, the mechanism by which R. solani infects crops. The candidate effectors trigging the host defence reaction, are expected to be applied in molecular breeding strategies to select the multiple resistant breeding materials. For the breeders, this is the cheapest and safest way to controlling the serious disease. Interestingly, resistant and sensitive rice materials can be selected through the potential effectors testing in our study. Hosts are now considered to be resistant to reported host-specific toxin effectors through the lack of dominant susceptibility genes and not through the presence of dominant resistance genes. However, the resistance/sensitivity mechanism of rice against R. solani AG1 IA is not clear. The effectors provide a fundamental tool for the investigation of the PHI, as well as vital information for the general characterization of necrotroph–plant interactions. Meanwhile, R. solani AG1 IA was also the first reported genome of the pathogen Rhizoctonia genus, it may serve as a model for studying the pathogenic mechanisms. R. solani AG1 IA isolates and culture conditions The R. solani AG1 IA strain was selected from a heavily infected rice plant from South China Agricultural University and was identified as the national standard isolate. The other isolates included in this study were selected from heavily infected rice plants in Sichuan Province and were used for further analyses. Based on the browning of the colony base, mycelial morphology, lactophenol cotton blue staining properties, the hyphal anastomosis and internal transcribed spacer test, 55 strains were selected and identified [5] ( Supplementary Note 1 ). The sequenced R. solani AG1 IA strain is a multinucleate diploid without the plasmids and hypovirulence. Its 13 chromosomes and 8–10 nuclei were observed ( Supplementary Fig. S1e ). The strain was grown in potato dextrose broth medium at 28 °C for 2 days in the dark with vigorous shaking (150 r.p.m.) and was then washed with sterile H 2 O, frozen in liquid N 2 and freeze dried, and genomic DNA was extracted using a modified CTAB method [5] , [7] . Genome sequencing and assembly Five libraries were constructed and sequenced using the Illumina GA II technology at the Beijing Genomics Institute ( Supplementary Table S1 ). Low-quality data that had a qual value of less than 20 and consisted of short reads (length<35 bp) were filtered from the raw data. The high-quality short reads were assembled using SOAPdenovo [10] . The heterozygosity and SNPs in the R. solani AG1 IA genome were analysed using the 173 and 347 bp library reads. Short reads were aligned to assembly sequence using the Burrows–Wheeler Aligner [42] . Then SNPs were calling using the SAMtools [43] mpileup and bcftools. Analysis of repeats De novo and homology analyses were employed to examine the repeats present in R. solani AG1 IA. PILER [44] and RepeatScout [45] were used for de novo detection. A de novo repeat library that included 81 families (74 RepeatScout families) was constructed. The results of the de novo method for repeat annotation was analysed using RepeatMasker v3-2-9 ( http://repeatmasker.org ). The homology analysis was performed using RepeatMasker with Repbase 16.09 (ref. 46 ). Gene prediction and annotation To obtain a more accurate gene set, we performed integrated prediction. Homologous proteins were identified through the Swiss-Prot database using BLAST v2.2.24. Novel candidate genes were obtained from running Augustus [47] and GeneMark-ES [48] , which were used as ab initio programs. To apply EuGene v3.6 (ref. 11 ) for integrated gene prediction, we obtained predicted translation start sites using NetStart [49] . Exon junctions were identified from RNA-seq using TopHat v1.1.4 (ref. 50 ). Using BLAST and HMMER v3.0 ( http://hmmer.janelia.org/ ), ORFs were annotated in the UniProt database, NCBI refseq fungi proteins and ORF domains were found in the Pfam database. Evolution OrthoMCL ( http://v2.orthomcl.org ) was used to identify ortholog, co-ortholog and inparalog pairs as well as reciprocal better hits for each pair. The pairs and their weights were used to construct the orthoMCL graph for clustering with the MCL algorithm [51] . To detect gene evolution rates, we calculated the tree branch lengths for 608 clusters of 1:1 orthologs of the ten fungi. The tree branch lengths indicated different evolutionary rates for these ortholog groups. The distribution of the branch length values was different from a normal distribution, as determined by the Shapiro–Wilk test ( P <0.01). Global alignment of the proteins of 608 ortholog groups with only one protein of one fungus was performed using CLUSTALW v2.1135 (ref. 52 ). Along with the phylogenetic tree of the ten fungi, we present the tree branch length of each ortholog group calculated using codeml with the JTT amino-acid substitution model from the PAML v4.4e package [53] . Transcriptome expression Fungal complementary DNA libraries were constructed from disease lesions at 10, 18, 24, 32, 48 and 72 h after inoculation, and each library product was sequenced using a library with a read insert size of 180 bp with Illumina GA II technology. We employed mRNA-Seq for expression analysis. The RNA expression analysis was based on the predicted genes of R. solani AG1 IA. First, Tophat [50] was used to map mRNA reads to the genome, and Cufflinks [54] was then used to calculate the expected fragments per kilobase of transcript per million fragments sequenced. Hierarchical clustering methods are applied to analyse gene expression data, and genes with similar functions group together [36] , [55] , [56] . Hierarchical clustering analysis of R. solani AG1 IA proteins were performed using transcriptome expression data (Correlation >0.98). Cluster v3.0 (ref. 57 ) was used to analyse the genome-wide expression data. Genes involved in pathogenicity and virulence-associated signalling pathway The CAZyme genes were identified using BLASTP with an e -value of less than 1e−50. The codes indicating the enzyme classes were those defined by the CAZyme database ( http://www.cazy.org/ ). The CAZymes database was from the CAZymes Analysis Toolkit (CAT) [58] . Using SMURF ( http://jcvi.org/smurf/run_smurf.php ) and NRPSpredictor [23] , the secondary metabolite genes were predicted. Cytochrome P450 genes are annotated in the P450 database with a threshold e -value of less than 1e−50 ( http://drnelson.uthsc.edu/cytochromeP450.html ). The ABC proteins were assigned to the ABC transporters in the UniProt database ( http://www.uniprot.org/ ) using BLASTP with an e -value≤8e−14 and the TCDB with an e -value ≤1e−50. The core elements of G-protein signalling pathway were predicted using BLASTP with a threshold e -value of less than 1e−50 ( http://www.genome.jp/kegg/pathway/sce/sce04011.html ). GPCRs were predicted based on a previous report [59] . The GPCR-like proteins were evaluated to verify the presence of seven transmembrane (7-TM) helices with TMPRED ( http://www.ch.embnet.org/software/TMPRED_form.html ), Phobius and TMHMM ( http://phobius.sbc.su.se/ , http://www.cbs.dtu.dk/services/TMHMM/ ). Secreted proteins The secreted proteins of R. solani AG1 IA were analysed using several prediction algorithms. SignalP3.0 ( http://www.cbs.dtu.dk/services/SignalP-3.0/ ) and Phobius ( http://phobius.binf.ku.dk/ ) were used to perform signal peptide cleavage site prediction. Transmembrane helices in the proteins were predicted using TMHMM ( http://www.cbs.dtu.dk/services/TMHMM-2.0/ ). Proteins located in the mitochondria, as determined by TargetP ( http://www.cbs.dtu.dk/services/TargetP/ ), were removed. The proteins that contained signal peptide cleavage sites and no transmembrane helices were selected as secreted proteins. GPI-anchored proteins were identified using big-PI ( http://mendel.imp.ac.at/gpi/fungi_server.html ). Candidate effectors and their validation Among the 145 genes encoding secreted proteins that showed a twofold or greater difference in expression during early infection progress in the rice–fungus interaction, we selected 45 candidate genes that had shown twofold or greater upregulation for verification of the function. These proteins, expressed by E. coli Transetta (DE3), were applied to rice, maize and soybean leaves, and we observed whether cell death phenotypes appeared in the leaves at 48 h post infiltration. All DNA manipulations and other procedures, including agarose gel electrophoresis, were performed according to standard protocols. The domains of these proteins were predicted based on annotation in the Pfam database ( http://pfam.sanger.ac.uk/ ). Hierarchical clustering was used to predict candidate effectors, which were predicted using Cluster (correlation >0.98) (ref. 55 ). Cluster v3.0 was used to analyse the genome-wide expression data. Among the 55 selected isolates, 13 and 2 intraspecific groups: R. solani AG1 IB and R. solani AG1 IC, were chosen for sequence analysis. The Codeml programme with models M0, M1, M2, M7 and M8 in PAML v4.4e package [53] was used for calculating dN/dS values and detecting positive selection. A neighbour-joining tree was produced based on the protein alignment using ClustalW v2.1, and protein distances were calculated using the PHYLIP ( http://evolution.genetics.washington.edu/phylip/ ) Protdist programme with the JTT model [60] . Expression vector construction and preparation A total of 45 expression plasmids were constructed with the pEASY-TlTM E1 Expression Vector (TransGen Biotech, Beijing, China). We obtained 45 complete genes from reverse-transcribed cDNA from a rice plant using PCR. Primers for these assays were designed based on our predicted gene sequences and included a Bam HI site and a Not I site. The obtained PCR products were gel-purified with a gel purification kit (AXYGen Biosciences, CA, USA) and cloned into the pEASY-TlTM E1 Expression vector. Total mycelial cDNA was obtained from the R. solani AG1 IA strain cultured in potato dextrose broth for 48 h using the RNAeasy Mini Kit (Qiagen, Hilden, Germany). After expressed in the E. coli strain Transetta (DE3) harbouring the pEASY-TlTM E1 vector, proteins were purified [32] . Toxin bioassay and fungal inoculation Toxin bioassays and fungal inoculation were conducted at the V11 phase rice leaf stage. Following fungal inoculation, the resultant disease was investigated according to the disease rating scale [8] . Three replicates of at least three plants of each line were evaluated in separate assays for toxin sensitivity and fungal inoculation. The fusion proteins were inoculated into detached leaves at 28 °C under 80% humidity. The leaves’ cell death phenotypes were observed after 48 h post infiltration. Data availability More detailed descriptions of the methods are provided in Supplementary Methods . All of the data generated in this project, including those related to genome assembly, gene prediction, gene functional annotations and transcriptomic data, may be accessed at the Sichuan Agricultural University (SICAU) official website: http://rice.sicau.edu.cn/sequence/fungi.zip . Accession codes: This Whole-Genome Shotgun project has been deposited at DDBJ/EMBL/GenBank under the accession code AFRT00000000. The version described in this paper is the first version, AFRT01000000. The transcriptome data accession codes are JP238634–JP285960. The transcriptome expression data from the six infection stages have been deposited under the following accessions codes: GSM807405–GSM807410. The fastq reads (SRA) are under accession codes SRX099909 and SRX099914 . How to cite this article: Zheng, A. et al . The evolution and pathogenic mechanisms of the rice sheath blight pathogen. Nat. Commun. 4:1424 doi: 10.1038/ncomms2427 (2013).